Hematopoietic PBX-interacting protein mediates cartilage degeneration during the pathogenesis of osteoarthritis Osteoarthritis (OA) has been recognized as the most common chronic age-related disease. Cartilage degeneration influences OA therapy. Here we report that hematopoietic pre-B cell leukemia transcription factor-interacting protein ( HPIP ) is essential for OA development. Elevated HPIP levels are found in OA patients. Col2a1-CreER T2 /HPIP f/f mice exhibit obvious skeletal abnormalities compared with their HPIP f/f littermates. HPIP deficiency in mice protects against developing OA. Moreover, intra-articular injection of adeno-associated virus carrying HPIP -specific short hairpin RNA in vivo attenuates OA histological signs. Notably, in vitro RNA-sequencing and chromatin immunoprecipitation sequencing profiles identify that HPIP modulates OA cartilage degeneration through transcriptional activation of Wnt target genes. Mechanistically, HPIP promotes the transcription of Wnt targets by interacting with lymphoid enhancer binding factor 1 ( LEF1 ). Furthermore, HPIP potentiates the transcriptional activity of LEF1 and acetylates histone H3 lysine 56 in the promoters of Wnt targets, suggesting that HPIP is an attractive target in OA regulatory network. Osteoarthritis (OA) is the most common worldwide age-related and post-traumatic degenerative joint disorder [1] , [2] , [3] . According to the statistics of the Centers for Disease Control and Prevention, arthritis affects an estimated 26.0% of women and 19.1% of men who are diagnosed by a doctor in the United States and OA is present in 80% of the population by age 65 [4] , [5] . OA is mainly characterized by a cartilage homeostasis disorder with subsequent inflammation and degradation that results in chronic physical disability and progressive irreversible dysfunction [6] , [7] , [8] , [9] . Although accumulating reports have identified factors to predict and modify the development of OA, the clinical efficacy of treatments for cartilage damage and regeneration is still very limited. Age, metabolism, and mechanical, genetic and environmental factors have gained widespread acceptance as the leading causes of degradation of cartilage extracellular matrix (ECM) molecules, such as collagen and aggrecan ( ACAN ), the loss of function of which is closely related to the progression of OA [10] , [11] , [12] . The maintenance of cartilage integrity and homeostasis depends on its normal structure and components [13] , [14] , [15] . Ultimately, this research will shed light on new therapies for the treatment of cartilage damage and degeneration in OA. Previously, we and others have shown that hematopoietic pre-B cell leukemia transcription factor-interacting ( PBX -interacting) protein ( HPIP/PBXIP1 ) mainly functions as a modulator of cancer carcinogenesis and progression [16] , [17] , [18] . HPIP silencing significantly suppresses migration/invasion and epithelial–mesenchymal transition (EMT) in lung cancer [19] . Stabilization of microtubules represses estrogen receptor α transcriptional activity in a HPIP -dependent manner [20] . The HPIP-ER complex network in breast cancer promotes cell proliferation and migration in vitro and in vivo [21] . Moreover, HPIP has also emerged as a novel substrate of calpain2 and activator of FAK [18] , which suggests the significance of HPIP in organogenesis and tumorigenesis. Besides, HPIP silencing suppressed TGF-β -induced EMT by inhibiting Smad2 activation and TGF-β treatment induced HPIP expression in cancer cells [22] , [23] . TGF-β is an endogenously pleiotropic cytokine that is known for the important regulation of OA cartilage homeostasis [6] . However, the potential role of HPIP in human OA remains unknown. In this study, using Col2a1-CreER T2 /HPIP f/f mice as an animal model, we find that HPIP is essential for the OA development. HPIP deficiency in chondrocyte-specific knockout of HPIP in mice protect against OA cartilage degeneration. Besides, intra-articular injection of adeno-associated virus (AAV) carrying HPIP -specific short hairpin RNA (shRNA) in vivo attenuates OA development. By combining RNA-sequencing (RNA-seq) and chromatin immunoprecipitation sequencing (ChIP-seq), we identify that HPIP modulates OA cartilage degeneration through transcriptional activation of Wnt signaling pathway and epigenetic modulation of transcriptional programs, suggesting that these novel functions of HPIP will likely lead to new avenues of OA treatment. Elevated HPIP levels in the cartilage of OA patients To investigate the potential role of HPIP in OA, we first examined the expression levels of HPIP in 118 pairs of OA cartilage tissues and corresponding non-lesion samples (Fig. 1a ). Prior to experimental assessment, we performed hematoxylin–eosin (HE), safranin O/fast green and Masson trichrome staining of the cartilage tissues of each patient (Fig. 1b ) and detected the expression of HPIP protein using an immunohistochemical staining assay and qRT-PCR in 118 pairs of OA cartilage tissues and corresponding non-lesion samples. HPIP expression was significantly higher in OA cartilage than in non-lesion tissues (Fig. 1c–d ). To further identify the stage of OA that HPIP expression manifests and assess the effects of the HPIP on the ECM components, we investigated the expression of HPIP and COL2A1 and ACAN at different stages of cartilage tissues using qRT-PCR analysis (Fig. 1e–g ). The data revealed that the expression of HPIP was gradually enhanced from stage 1 and the sustainable increase in the mRNA levels of the HPIP was significantly observed in stage 4 of OA cartilage, whereas the production of COL2A1 and ACAN decreased gradually from stage 1 to the late stage of OA, indicating the potential involvement of HPIP in ECM degradation in OA articular cartilage degeneration. Fig. 1 HPIP expression is upregulated in osteoarthritis (OA) cartilage. a Representative plain radiographs and MRI images of patients with knee OA undergoing knee arthroplasty surgery. A–P anterior–posterior. b Representative histopathological staining of normal and OA cartilage tissues. Hematoxylin–eosin, safranin O/fast green and Masson trichrome staining were performed to examine the proteoglycan content in cartilage. Scale bar, left, 500 μm; right, 200 μm. c Immunohistochemistry assay with anti- HPIP in normal and OA cartilage tissues. Scale bar, left, 500 μm; right, 50 μm. d The HPIP scores in normal ( n = 118) and OA ( n = 118) cartilage tissues based on an immunohistochemistry assay were compared with the Mann–Whitney U -test. Center value represents the median of the HPIP scores. The bounds of box represent the upper quartile and the lower quartile. The whiskers represent the maximum and minimum score. e qRT-PCR measurement of HPIP in cartilage tissues obtained from stage 0 (S0) to stage 4 (S4). f qRT-PCR measurement of COL2A1 in cartilage tissues obtained from stage 0 (S0) to stage 4 (S4). g qRT-PCR measurement of ACAN in cartilage tissues obtained from stage 0 (S0) to stage 4 (S4). Error bar represents the standard deviation (s.d.) and P- value was generated by using one-way ANOVA with Tukey’s post hoc test. * P < 0.05; ** P < 0.01 Full size image HPIP deficiency impaired articular cartilage development To determine the physiological involvement of endogenous HPIP gene in cartilage homeostasis, we next investigated the phenotype of chondrocyte-specific HPIP knockout (KO) mice. Pregnant mice with embryos at E12.5 were injected with tamoxifen. The knockdown efficiency of HPIP was confirmed by DNA sequencing and immunoblot in Col2a1-CreER T2 /HPIP f/f mice (Supplementary Fig. 1a, b ). Whole skeletal alizarin red, alcian blue staining, μCT and HE staining were performed. The Col2a1-CreER T2 /HPIP f/f mice showed mild but proportional dwarfism compared to HPIP f/f littermates from embryonic stages up to 1 week after birth (Fig. 2a–c and Supplementary Fig. 2a ). The lengths of the humerus, radius, ulna, femur, tibia, and vertebrae were 10–21% shorter in Col2a1-CreER T2 /HPIP f/f mice than in their HPIP f/f littermates (Fig. 2d ). In addition, we also investigated the skeletal phenotype of HPIP complete knockout mice, the HPIP complete knockout mice also showed proportional dwarfism than the wild-type littermates (Supplementary Fig. 2b,c ). Moreover, the histological assays indicated that within the total limb of Col2a1-CreER T2 /HPIP f/f mice, the percentage of the proliferative zone was moderately increased, indicating abnormal hypertrophic differentiation caused by HPIP insufficiency. The percentage of the hypertrophic zone was also increased while that of the bone zone was decreased in the limbs of Col2a1-CreER T2 /HPIP f/f mice, suggesting that HPIP insufficiency affected not only chondrocyte hypertrophy but also subsequent steps, such as matrix degradation (Fig. 2e and Supplementary Fig. 1c ). We then performed immunohistochemical staining, qRT-PCR and western blotting to detect the expression of the cartilage matrix components COL2A1 , ACAN , and COLX . The results confirmed that COL2A1 and ACAN expression was suppressed, whereas COLX expression was increased in the articular joint of Col2a1-CreER T2 /HPIP f/f mice compared with that of their HPIP f/f littermates (Fig. 2f, g and Supplementary Fig. 1d–f ). Fig. 2 Skeletal and cartilage abnormalities in Col2a1-CreER T2 ;HPIP f/f mice. a Col2a1-CreER T2 ;HPIP f/f mice and HPIP f/f littermate embryos (P1). Scale bar, 1 mm. b Double staining with alizarin red and alcian blue of the whole skeleton. Scale bar, 1 mm. c Lateral and posterior–anterior (P–A) views of μCT three-dimensional reconstruction analysis. Scale bar, 1 mm. d The length of long bones and vertebra (first to fifth lumbar spines) of HPIP f/f ( n = 10) and Col2a1-CreER T2 ;HPIP f/f ( n = 10) littermate embryos (P1). e Masson trichrome staining of whole tibias. The boxed areas represent the regions of right magnified images with a matched color rim. Scale bar, 100 μm. The percentage of the length of the proliferative zone (blue), hypertrophic zone (red), and bone area (gray) over the total tibia length of HPIP f/f ( n = 10) and Col2a1-CreER T2 ;HPIP f/f ( n = 10) littermate embryos (P1). f , g Representative immunohistochemistry assay ( f ) with the indicated antibodies of the proximal tibias of HPIP f/f and Col2a1-CreER T2 ;HPIP f/f littermate embryos (P1) and boxplots showing qRT-PCR ( g ) of the proximal tibias of HPIP f/f ( n = 10) and Col2a1-CreER T2 ;HPIP f/f ( n = 10) littermate embryos (P1). Scale bar, 100 μm. Center value represents the median of the HPIP scores. The bounds of box represent the upper quartile and the lower quartile. The whiskers represent the maximum and minimum score. Error bar represents the standard deviation (s.d.) and P- value was generated by using one-way ANOVA with Tukey’s post hoc test. * P < 0.05; ** P < 0.01 Full size image Ablation of HPIP prevents OA development Next, we investigated the function of HPIP in OA pathogenesis. At 8 weeks, plain radiographs and histomorphometric analyses and μCT showed that the size of the knee in Col2a1-CreER T2 /HPIP f/f had no significant difference with the HPIP f/f littermates (Fig. 3a and Supplementary Fig. 3a, b ). Because HPIP was shown to function as a corepressor of PBX1 and PBX1 has a role in osteogenesis [24] , we then detected the expression of PBX1 and bone characteristics of bone volume fraction, tissue mineral density, connectivity density, trabecular separation, and trabecular thickness in the Col2a1-CreER T2 /HPIP f/f and HPIP f/f littermates to identify whether the phenotype of the Col2a1-CreER T2 /HPIP f/f mice was in fact due to increased activity of PBX1 . The results revealed that the expression of PBX1 was enhanced in Col2a1-CreER T2 /HPIP f/f mice. Besides, further analysis showed that an increased bone volume fraction, tissue mineral density, connectivity density, and trabecular thickness while a reduction trabecular separation in Col2a1-CreER T2 /HPIP f/f mice compared with those of HPIP f/f littermates (Supplementary Fig. 3c–h ). Then, Col2a1-CreER T2 /HPIP f/f mice and their HPIP f/f littermates underwent surgery to perform anterior cruciate ligament transection (ACLT) in their knee joints. The cartilage thickness and bone area covered by cartilage in mice after surgical transection were examined by histopathological analyses and μCT (Supplementary Fig. 3i, j and Supplementary Table 2 ). 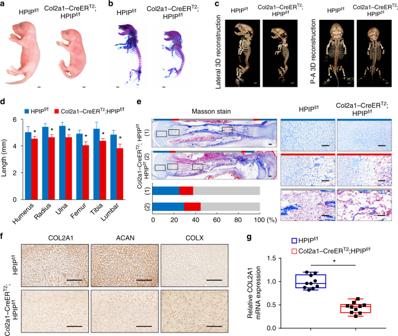Fig. 2 Skeletal and cartilage abnormalities inCol2a1-CreERT2;HPIPf/fmice.aCol2a1-CreERT2;HPIPf/fmice andHPIPf/flittermate embryos (P1). Scale bar, 1 mm.bDouble staining with alizarin red and alcian blue of the whole skeleton. Scale bar, 1 mm.cLateral and posterior–anterior (P–A) views of μCT three-dimensional reconstruction analysis. Scale bar, 1 mm.dThe length of long bones and vertebra (first to fifth lumbar spines) ofHPIPf/f(n= 10) andCol2a1-CreERT2;HPIPf/f(n= 10) littermate embryos (P1).eMasson trichrome staining of whole tibias. The boxed areas represent the regions of right magnified images with a matched color rim. Scale bar, 100 μm. The percentage of the length of the proliferative zone (blue), hypertrophic zone (red), and bone area (gray) over the total tibia length ofHPIPf/f(n= 10) andCol2a1-CreERT2;HPIPf/f(n= 10) littermate embryos (P1).f,gRepresentative immunohistochemistry assay (f) with the indicated antibodies of the proximal tibias ofHPIPf/fandCol2a1-CreERT2;HPIPf/flittermate embryos (P1) and boxplots showing qRT-PCR (g) of the proximal tibias ofHPIPf/f(n= 10) andCol2a1-CreERT2;HPIPf/f(n= 10) littermate embryos (P1). Scale bar, 100 μm. Center value represents the median of theHPIPscores. The bounds of box represent the upper quartile and the lower quartile. The whiskers represent the maximum and minimum score. Error bar represents the standard deviation (s.d.) andP-value was generated by using one-way ANOVA with Tukey’s post hoc test. *P< 0.05; **P< 0.01 Before sham surgery, Col2a1-CreER T2 /HPIP f/f mice revealed similar articular cartilage thickness and areas compared with their HPIP f/f littermates. However, HPIP f/f mice showed lower cartilage thickness and covered cartilage areas compared with Col2a1-CreER T2 /HPIP f/f mice at 4 and 8 weeks after transection (Fig. 3b and Supplementary Table 2 ). The OARSI histological grading scale of articular cartilage revealed that Col2a1-CreER T2 /HPIP f/f mice scored lower than their HPIP f/f littermates (Fig. 3b ). In addition, histopathological analysis showed that Col2a1-CreER T2 /HPIP f/f mice displayed less severe OA cartilage degradation (Supplementary Fig. 3k ). Furthermore, we assessed the structure of tibial subchondral bone using μCT. The result found improvement of trabeculae connectivity and microarchitecture in Col2a1-CreER T2 /HPIP f/f mice relative to HPIP f/f littermates at 4 and 8 weeks after transection, as demonstrated by the normalization of subchondral bone tissue volume and a lower trabecular pattern factor (Supplementary Fig. 3l, m ). Besides the immunohistochemical staining assay and qRT-PCR confirmed decreased expression of COL2A1 and ACAN in noncalcified cartilage of HPIP f/f mice compared with that of Col2a1-CreER T2 /HPIP f/f mice (Fig. 3c, d ). Moreover, HPIP deficiency significantly reduced mRNA levels of inflammatory markers, such as IL-1β , TNF-α , MMP-13 , and ADAMTS5 according to the qRT-PCR analysis (Supplementary Fig. 3n ). The progression of OA is accompanied by secondary clinical symptoms. Rotarod and hotplate analysis and pain measurement showed that HPIP f/f mice had an increased hotplate response time and decreased rotarod time, weight bearing and distance traveled, whereas Col2a1-CreER T2 /HPIP f/f mice with or without transection revealed no significant differences in rotarod or hotplate response times or weight bearing and distance traveled (Fig. 3e–g ), thus suggesting HPIP ablation prevents OA progression. Fig. 3 HPIP ablation protects mice from the progression of osteoarthritis (OA). a Plain radiographs of the entire body (left) and knee (right) of the HPIP f/f and Col2a1-CreER T2 ;HPIP f/f littermates (8 weeks old). Scale bar: 10 mm (left), 1 mm (right). b Quantitative analysis of the covered surface area and OARSI grade in mice ( n = 10). c Immunohistochemistry assay with the indicated antibodies in mice 8 weeks after ACLT. Scale bar, 100 μm. d qRT-PCR examination of COL2A1 and ACAN in HPIP f/f and Col2a1-CreER T2 ;HPIP f/f littermate (8 weeks after ACLT). e Time of mice on the rotarod 8 weeks after ACLT and the response time of mice in the hotplate analysis ( n = 10). f Difference in hind paw weight bearing ( g ) in mice (8 weeks old) after ACLT ( n = 10). g Traveled distance per 6 min in an open field, in mice after ACLT ( n = 10). Data are expressed as the means ± standard deviation. h Scheme of the OA treatment with adeno-associated virus (AAV) carrying HPIP -specific shRNA in mice. i Safranin O/fast green staining of whole tibias of mice. Two weeks after surgery, C57/BL6J mice (8 weeks old) were injected intra-articularly with AAV carrying HPIP -specific shRNA and analyzed 6 weeks later. ( j ) The OARSI grades of the mice are shown ( n = 10). Scale bar, 250 μm. Cs Control shRNA; Hs HPIP shRNA. Sg Surgery. k Sagittal views of μCT and three-dimensional images of the knee joints. Scale bar, 1 mm. Quantitative analysis of the cartilage surface area is shown ( n = 10). Error bar represents the standard deviation (s.d.) and P value was generated by using one-way ANOVA with Tukey’s post hoc test. Cs Control shRNA; Hs HPIP shRNA. Sg Surgery. * P < 0.05; ** P < 0.01 Full size image Gene transfer with HPIP -specific shRNA treats OA To further investigate the role of HPIP in OA treatment, 8-week-old C57BL/6J wild-type mice underwent ACLT surgery. 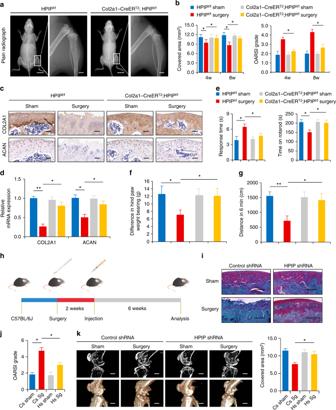Fig. 3 HPIPablation protects mice from the progression of osteoarthritis (OA).aPlain radiographs of the entire body (left) and knee (right) of theHPIPf/fandCol2a1-CreERT2;HPIPf/flittermates (8 weeks old). Scale bar: 10 mm (left), 1 mm (right).bQuantitative analysis of the covered surface area and OARSI grade in mice (n= 10).cImmunohistochemistry assay with the indicated antibodies in mice 8 weeks after ACLT. Scale bar, 100 μm.dqRT-PCR examination ofCOL2A1andACANinHPIPf/fandCol2a1-CreERT2;HPIPf/flittermate (8 weeks after ACLT).eTime of mice on the rotarod 8 weeks after ACLT and the response time of mice in the hotplate analysis (n= 10).fDifference in hind paw weight bearing (g) in mice (8 weeks old) after ACLT (n= 10).gTraveled distance per 6 min in an open field, in mice after ACLT (n= 10). Data are expressed as the means ± standard deviation.hScheme of the OA treatment with adeno-associated virus (AAV) carryingHPIP-specific shRNA in mice.iSafranin O/fast green staining of whole tibias of mice. Two weeks after surgery, C57/BL6J mice (8 weeks old) were injected intra-articularly with AAV carryingHPIP-specific shRNA and analyzed 6 weeks later. (j) The OARSI grades of the mice are shown (n= 10). Scale bar, 250 μm. Cs Control shRNA; HsHPIPshRNA. Sg Surgery.kSagittal views of μCT and three-dimensional images of the knee joints. Scale bar, 1 mm. Quantitative analysis of the cartilage surface area is shown (n= 10). Error bar represents the standard deviation (s.d.) andPvalue was generated by using one-way ANOVA with Tukey’s post hoc test. Cs Control shRNA; HsHPIPshRNA. Sg Surgery. *P< 0.05; **P< 0.01 Two weeks after transection, an intra-articular injection of AAV encoding HPIP -specific shRNA was performed (Fig. 3h ). The efficiency of AAV encoding HPIP -specific shRNA in the joints was evaluated by immunohistochemical staining assay and western blotting and qRT-PCR (Supplementary Fig. 4a–c ). Mice that did not receive the injection of HPIP -specific shRNA showed more severe OA cartilage degradation, a higher OARSI grade and increased tibial subchondral bone tissue volume and trabecular pattern factor, and a lower cartilage thickness and covered cartilage area compared with mice that received the injection (Fig. 3h–k and Supplementary Fig. 4d–g ). Moreover, we also found a decreased expression of COL2A1 and ACAN and increased expression of IL-1β , TNF-α , MMP-13 , and ADAMTS5 in the cartilage of mice that did not receive the HPIP -specific shRNA treatment (Supplementary Fig. 4h–j ). Taken together, these data demonstrate that HPIP inhibition with HPIP -specific shRNA protects the joints from OA cartilage impairment. RNA-seq analysis of downstream genes regulated by HPIP We then examined HPIP -mediated transcriptional targets that could account for cartilage degeneration during the pathogenesis of OA. 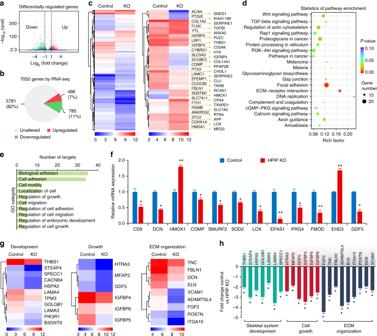Fig. 4 RNA-seq analysis ofHPIP-modulated genes.aA volcano plot illustrating differentially regulated gene expression from RNA-seq analysis between the control andHPIPknockout (KO) chondrocytes. Genes upregulated and downregulated are shown in red and green, respectively. Values are presented as the log2 of tag counts.bRNA-seq comparison revealed a total of 7052 genes expressed, of which 486 genes were upregulated and 785 genes were downregulated.cThe hierarchical clustering of the RNA-seq analysis results shows all genes that were significantly different expressed (left panel) and the representative top 50 genes that were differentially expressed (right panel).dKEGG pathway analysis of downregulated targets inHPIP-deficient transcriptome.egene ontology (GO) functional clustering of genes that were downregulated for biological processes. (The top 10 most significantly affected categories are shown).fqRT-PCR validation analysis of the indicated genes regulated byHPIP.gHeatmap of representative cartilage development, growth, and extracellular matrix (ECM) organization-related genes.hqRT-PCR validation analysis shows the mRNA expression fold change of skeletal system development, cell growth and ECM organization-associated genes in the control vsHPIPKO chondrocytes. Error bar represents the standard deviation (s.d.) andP-value was generated by using one-way ANOVA with Tukey’s post hoc test. *P< 0.05; **P< 0.01 RNA-seq analysis was performed in HPIP KO and the control chondrocytes. Before the RNA-seq analysis, the KO efficiency of HPIP in chondrocytes was confirmed by western blotting (Supplementary Fig. 5a ). Among the 1271 significantly differentially expressed genes (DEGs), transcripts of 486 (7%) genes were upregulated, whereas transcripts of 785 (11%) genes including COL2A1 ( P = 3.57 × 10 −5 , fold difference = −3.3084) were downregulated in HPIP KO compared to the control chondrocytes (Fig. 4a, b ). The representative top 50 most significant genes with altered expression are shown (Fig. 4c and Supplementary Fig. 5b–e and Supplementary Tables 3 and 4 ). In addition, gene ontology (GO) enrichment analysis demonstrated significantly affected categories in genes that were downregulated or upregulated in response to HPIP deficiency. The downregulated genes were associated with ECM structural constituents (GO: 0031012, 0044420, 0005578) and the extracellular region (GO: 0005576, 0044421) (Fig. 4e and Supplementary Fig. 6a, b and Supplementary Table 5 ). 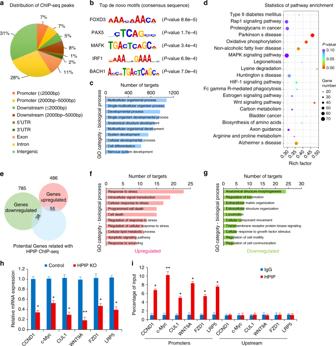Fig. 5 Chromatin immunoprecipitation (ChIP) analysis of cartilage homeostasis-related genes regulated byHPIP.aHPIP-binding regions are mapped by ChIP-seq. The annotation shows that a peak is in the promoter (defined as ≤2000 bp), the promoter (defined as 2000–5000 bp), downstream of the promoter (defined as ≤2000 bp), downstream of the promoter (defined as 2000–5000 bp), 5′ UTR, 3′ UTR, intron or intergenic.bTop de novo motifs enriched in the vicinity of theHPIP-binding sites.cGO functional clustering of targets associated withHPIPChIP-seq peaks for biological process (top 10 most significantly affected categories are shown).dKEGG pathway enrichment analysis of targets associated withHPIPChIP-seq peaks.eAn overlay of RNA-seq and ChIP-seq analysis results revealed genes as potential direct targets ofHPIPin chondrocytes.f,gGene ontology (GO) functional clustering of genes that were upregulated and downregulated for identification of biological processes directly regulated byHPIP, respectively (top 10 categories most significantly affected are shown).hqRT-PCR validation analysis of the indicated genes in the control vsHPIPKO chondrocytes.iChIP assay forHPIPoccupancy on theCCND1,c-Myc,CUL1,WNT9A,FZD1, andLRP5promoters or upstream of the promoters in chondrocytes. Error bar represents the standard deviation (s.d.) andP-value was generated by using one-way ANOVA with Tukey’s post hoc test. *P< 0.05; **P< 0.01 Upregulated GO terms indicating amino acid transport (GO: 0003333, 0006865), cell cycle arrest (GO: 0007050) and cell death (GO: 0010941), combined with pathway analysis results of glutathione metabolism and apoptosis (Supplementary Fig. 6c-f and Supplementary Table 6 ), suggesting that HPIP is closely involved in chondrocyte homeostasis. 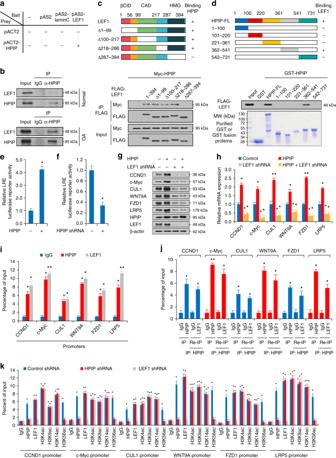Fig. 6 HPIPacetylatesH3K56acat the promoters ofWnttarget genes.aYeast CG1945 cells were transformed with the indicated plasmids (bait and prey for the two-hybrid assay) and grown on selective media. Positive interaction is indicative of colonies that grow on selective media and have β-galactosidase activity.bNormal or osteoarthritis (OA) chondrocytes were immunoprecipitated with anti-HPIPor normal IgG, and the precipitates were analyzed by immunoblot with the indicated antibodies. IP immunoprecipitation.cThe top panel shows a schematic diagram of theLEF1fragments used to map the interaction withHPIP. Δ deficient fragment, βCIDβ-catenininteraction domain, CAD context-dependent activation domain, HMG high-mobility group domain. Cell lysates of theLEF1fragments were IP with the indicated antibodies.dThe top panel shows a schematic diagram of theHPIPfragments used to map the interaction withLEF1. Immunoblot analysis of bound proteins in lysates of OA chondrocytes expressingFLAG-LEF1following incubation with Sepharose beads coupled toGSTalone or variousGST-HPIPfusion proteins.e,fLuciferase assay in cultured chondrocytes infected withLEF1-response element (LRE) reporter andHPIP(e) orHPIPshRNA (f).gCultured human chondrocytes were infected with the HPIP plasmid and the vector control or shRNA forLEF1. Immunoblots were incubated with the indicated antibodies.hqRT-PCR analysis of the indicated group.iChIP analysis ofHPIPandLEF1occupancy on the indicatedWnttarget gene promoters.jRe-ChIP analysis of the occupancy ofHPIPandLEF1on the indicatedWnttarget gene promoters.kChIP analysis ofHPIP,LEF1, and histone H3 acetylation occupancy on the indicatedWnttarget gene promoters inHPIPorLEF1knockdown chondrocytes. Error bar represents the standard deviation (s.d.) andP-value was generated by using one-way ANOVA with Tukey’s post hoc test. *P< 0.05; **P< 0.01 As RNA-seq analysis indicated the altered expression of genes related to cell adhesion which is supported by previous findings that were attributed to HPIP functions, we then performed cell adhesion and migration assay to investigate the function of HPIP . The results revealed that HPIP deficiency inhibited cell adhesion and migration in chondrocytes (Supplementary Fig. 6g, h ). Furthermore, KEGG pathway analysis showed that DNA replication, the ECM–receptor interaction and Wnt signaling pathways were downregulated, whereas the p53 signaling pathway was upregulated in HPIP KO chondrocytes (Fig. 4d and Supplementary Fig. 6f and Supplementary Tables 7 and 8 ). Among the 1271 significantly DEGs regulated by HPIP , over 400 genes have previously been reported to be associated with OA. We then performed qRT-PCR to examine the representative 12 genes mediated by HPIP (Fig. 4f ). The results indicated that HMOX1 and EHD3 were upregulated in HPIP KO chondrocytes, whereas genes such as CD9 , DCN , SMURF2 , GDF5 , and so on were downregulated in HPIP KO chondrocytes (Fig. 4f ). Moreover, many of the DEGs are crucial for development, growth and ECM organization (Fig. 4g ). We then validated the differentially altered targets using qRT-PCR. Consistent with the RNA-seq data, qRT-PCR confirmed the mRNA expression of the targets (Fig. 4h ). Taken together, these data reveal that HPIP acts as a crucial regulator in OA articular cartilage homeostasis. Fig. 4 RNA-seq analysis of HPIP -modulated genes. a A volcano plot illustrating differentially regulated gene expression from RNA-seq analysis between the control and HPIP knockout (KO) chondrocytes. Genes upregulated and downregulated are shown in red and green, respectively. Values are presented as the log2 of tag counts. b RNA-seq comparison revealed a total of 7052 genes expressed, of which 486 genes were upregulated and 785 genes were downregulated. c The hierarchical clustering of the RNA-seq analysis results shows all genes that were significantly different expressed (left panel) and the representative top 50 genes that were differentially expressed (right panel). d KEGG pathway analysis of downregulated targets in HPIP -deficient transcriptome. e gene ontology (GO) functional clustering of genes that were downregulated for biological processes. (The top 10 most significantly affected categories are shown). f qRT-PCR validation analysis of the indicated genes regulated by HPIP . g Heatmap of representative cartilage development, growth, and extracellular matrix (ECM) organization-related genes. h qRT-PCR validation analysis shows the mRNA expression fold change of skeletal system development, cell growth and ECM organization-associated genes in the control vs HPIP KO chondrocytes. Error bar represents the standard deviation (s.d.) and P- value was generated by using one-way ANOVA with Tukey’s post hoc test. * P < 0.05; ** P < 0.01 Full size image ChIP-seq analysis of direct transcriptional targets of HPIP To further explore the underlying molecular mechanisms of HPIP -mediated OA cartilage degeneration and assess the direct downstream transcriptional targets of HPIP , we performed a genome-wide ChIP-seq assay. The ChIP-seq data were examined by a quality evaluation (Supplementary Fig. 7 ). The results demonstrated that of 3136 significant ChIP-seq peaks for HPIP , including PBX1 (Fig. 5a and Supplementary Fig. 8a ). De novo motif analysis suggested that the most highly enriched DNA-binding motifs among HPIP -bound regions occurred in the FOXD3 , PAX5 , MAFK , IRF1 , and BACH1 genes (Fig. 5b ), indicating that these transcription factors may act as effector factors of HPIP . Besides, GO analysis revealed that these targets were involved in crucial organism processes, cell differentiation and the extracellular matrix (Fig. 5c and Supplementary Fig. 8b, c and Supplementary Table 9 ). Moreover, KEGG pathway analysis showed potential targets involved in Parkinson’s disease, oxidative phosphorylation and the Wnt signaling pathway (Fig. 5d ). We then analyzed the intersection of the ChIP-seq and RNA-seq data and found that 93 targets were directly regulated by HPIP deficiency (Fig. 5e ). GO analysis of the direct targets of HPIP deficiency indicated that the upregulated categories included intracellular signal transduction and protein kinase activity (Fig. 5f and Supplementary Fig. 8d, e ), whereas the downregulated categories due to HPIP deficiency were highly enriched for anatomical structure morphogenesis and extracellular matrix organization (Fig. 5g and Supplementary Fig. 8f, g ), which are in line with the results of RNA-seq. We then validated the altered expression of a subset of targets from the intersection of the ChIP-seq and RNA-seq data using qRT-PCR. The results confirmed that the mRNA expression levels of the downstream targets of the Wnt signaling pathway ( CCND1 , c-Myc , CUL1 , WNT9A , FZD1, and LRP5 ) were significantly downregulated in HPIP -deficient chondrocytes (Fig. 5h ). Furthermore, ChIP analysis found a significant enrichment of HPIP in the Wnt target gene promoter regions (Fig. 5i ). Therefore, we focused on the Wnt signaling pathway to decipher the molecular network around HPIP in OA cartilage degeneration. Fig. 5 Chromatin immunoprecipitation (ChIP) analysis of cartilage homeostasis-related genes regulated by HPIP . a HPIP -binding regions are mapped by ChIP-seq. The annotation shows that a peak is in the promoter (defined as ≤2000 bp), the promoter (defined as 2000–5000 bp), downstream of the promoter (defined as ≤2000 bp), downstream of the promoter (defined as 2000–5000 bp), 5′ UTR, 3′ UTR, intron or intergenic. b Top de novo motifs enriched in the vicinity of the HPIP -binding sites. c GO functional clustering of targets associated with HPIP ChIP-seq peaks for biological process (top 10 most significantly affected categories are shown). d KEGG pathway enrichment analysis of targets associated with HPIP ChIP-seq peaks. e An overlay of RNA-seq and ChIP-seq analysis results revealed genes as potential direct targets of HPIP in chondrocytes. f , g Gene ontology (GO) functional clustering of genes that were upregulated and downregulated for identification of biological processes directly regulated by HPIP , respectively (top 10 categories most significantly affected are shown). h qRT-PCR validation analysis of the indicated genes in the control vs HPIP KO chondrocytes. i ChIP assay for HPIP occupancy on the CCND1 , c-Myc , CUL1 , WNT9A , FZD1 , and LRP5 promoters or upstream of the promoters in chondrocytes. Error bar represents the standard deviation (s.d.) and P- value was generated by using one-way ANOVA with Tukey’s post hoc test. * P < 0.05; ** P < 0.01 Full size image HPIP stimulates Wnt signaling by interacting with LEF1 Interactions of transcription factors with genes are closely associated with active transcription. To investigate how HPIP regulates Wnt target gene transcription, we used the Yeast Two Hybrid System combined with coimmunoprecipitation (Co-IP) to identify its interaction partners. The Yeast Two Hybrid experiment revealed that the transcription factor LEF1 physically interacted with HPIP (Fig. 6a ). CO-IP of endogenous proteins confirmed the HPIP/LEF1 interaction in chondrocytes (Fig. 6b ). As LEF1 was a good partner of β-catenin , we performed subcellular separation combined with immunoprecipitation assay to investigate the role of β-catenin involved in HPIP/LEF1 complex. The results revealed that HPIP was located in both nucleus (32%) and cytoplasm (68%) in chondrocytes. Endogenous HPIP interacted with endogenous β-catenin , from both cytoplasmic and nuclear fractions of cells. Endogenous HPIP or β-catenin associated with endogenous LEF1 in the nucleus (Supplementary Fig. 9a ). Next, we performed the immunofluorescence analysis and found HPIP could be colocalized with LEF1 in the nucleus (Supplementary Fig. 9b ). More importantly, β-catenin knockdown significantly diminished the physical interaction between HPIP and LEF1 , indicating that the interaction of HPIP and LEF1 is mediated by β-catenin (Supplementary Fig. 9c ). We then examined the region of LEF1 that interacts with HPIP using synthesized LEF1 deletions and a CO-IP assay (Fig. 6c ). All of the deletions from the N terminus of LEF-1 (Δ1–99, Δ100–217 and Δ218–286) retained the ability to interact with HPIP , whereas removal of the high mobility group (HMG) domain of LEF1 (Δ287–394) eliminated the interaction with HPIP (Fig. 6c ), suggesting that the interactions are localized to the LEF-1 HMG domain. Fig. 6 HPIP acetylates H3K56ac at the promoters of Wnt target genes. a Yeast CG1945 cells were transformed with the indicated plasmids (bait and prey for the two-hybrid assay) and grown on selective media. Positive interaction is indicative of colonies that grow on selective media and have β-galactosidase activity. b Normal or osteoarthritis (OA) chondrocytes were immunoprecipitated with anti- HPIP or normal IgG, and the precipitates were analyzed by immunoblot with the indicated antibodies. IP immunoprecipitation. c The top panel shows a schematic diagram of the LEF1 fragments used to map the interaction with HPIP . Δ deficient fragment, βCID β-catenin interaction domain, CAD context-dependent activation domain, HMG high-mobility group domain. Cell lysates of the LEF1 fragments were IP with the indicated antibodies. d The top panel shows a schematic diagram of the HPIP fragments used to map the interaction with LEF1 . Immunoblot analysis of bound proteins in lysates of OA chondrocytes expressing FLAG-LEF1 following incubation with Sepharose beads coupled to GST alone or various GST-HPIP fusion proteins. e , f Luciferase assay in cultured chondrocytes infected with LEF1 -response element (LRE) reporter and HPIP ( e ) or HPIP shRNA ( f ). g Cultured human chondrocytes were infected with the HPIP plasmid and the vector control or shRNA for LEF1 . Immunoblots were incubated with the indicated antibodies. h qRT-PCR analysis of the indicated group. i ChIP analysis of HPIP and LEF1 occupancy on the indicated Wnt target gene promoters. j Re-ChIP analysis of the occupancy of HPIP and LEF1 on the indicated Wnt target gene promoters. k ChIP analysis of HPIP , LEF1 , and histone H3 acetylation occupancy on the indicated Wnt target gene promoters in HPIP or LEF1 knockdown chondrocytes. Error bar represents the standard deviation (s.d.) and P- value was generated by using one-way ANOVA with Tukey’s post hoc test. * P < 0.05; ** P < 0.01 Full size image Next, we performed GST pull-down experiments to identify the region of HPIP that interacts with LEF1 (Fig. 6d ). The results showed that the FLAG-tagged LEF1 protein interacted with purified GST- HPIP , but not GST alone (Fig. 6d ). Besides, we noticed that the molecular weight of HPIP (1–100) was little larger than that was predicted by the sequence data, which might be caused by posttranslational modifications because its coding sequence and open reading frame was correct according to the DNA sequencing results. Importantly, we found that HPIP (362–541), but not other HPIP regions (1–100, 101–200, 221–361, 542–731), was associated with HPIP (Fig. 6d ), indicating that region 362–541 is necessary for the HPIP–LEF1 interaction. HPIP acetylates H3K56ac at the promoters of Wnt target genes Next, we examined how HPIP regulates Wnt target gene transcription in OA. We first performed a luciferase reporter assay that revealed that the luciferase activity of LEF1 -response element (LRE) was significantly increased by introduction of HPIP into chondrocytes (Fig. 6e ), whereas inhibition of HPIP diminished this activity (Fig. 6f ), suggesting that HPIP might promote Wnt signaling activation through LEF1 . We then examined whether LEF-1 is required for HPIP -mediated expression of Wnt target genes. The results showed that HPIP overexpression increased the expression of Wnt targets ( CCND1 , c-Myc , CUL1 , WNT9A , FZD1, and LRP5 ), whereas knockdown of endogenous LEF-1 inhibited the expression of Wnt targets ( CCND1 , c-Myc , CUL1 , WNT9A , FZD1, and LRP5 ) and abolished the ability of HPIP to modulate Wnt target production (Fig. 6g, h ), indicating that LEF1 is important for HPIP -mediated Wnt target gene expression regulation. Furthermore, the ChIP assay revealed that like HPIP , LEF1 was recruited to the HPIP -binding sites of the CCND1 , c-Myc , CUL1 , WNT9A , FZD1 , and LRP5 promoters in chondrocytes (Fig. 6i ). Re-ChIP experiments showed that HPIP was associated with LEF1 on the corresponding binding sites (Fig. 6j ). Because the histone acetylation regulated by histone acetyltransferases is often associated with active transcription of genes, we then investigated whether HPIP regulates Wnt target expression via modification of the chromatin status in chondrocytes. LEF1 knockdown reduced the recruitment of HPIP and acetylation of H3K56ac , but not H3K4ac , H3K9ac or H3K14ac , to the promoters of CCND1 , c-Myc , CUL1 , WNT9A , FZD1, and LRP5 in chondrocytes (Fig. 6k ). HPIP inhibition also caused marked suppression of recruitment of H3K56ac , but not H3K4ac , H3K9ac , and H3K14ac , to the HPIP/LEF1 binding sites, indicating that H3K56ac activity is important for HPIP modulation of gene transcription. Site specificity of histone is mainly determined by distinct types of histone acetyltransferases (HATs) complex. To further investigate how HPIP/LEF1 complex specifically promotes H3K56ac , we searched for the potential HATs in HPIP -preying proteins screened out by Yeast Two Hybrid assay and found two HATs, p300 and GCN5 as the potential HPIP/LEF1 partners. Co-IP assay further confirmed that acetyltransferase p300 , acetylating H3K56 site, rather than GCN5 [25] ,, acetylating H3K4 , H3K9 , and H3K14 sites, specifically interacted with HPIP , which might explain for the site acetylation preference of the histone (Supplementary Fig. 9d, e ). We next evaluated the proliferative activities of LEF1 and HPIP in chondrocytes using cell growth assays. In line with the above results, HPIP or LEF1 inhibition suppressed the proliferation of chondrocytes (Supplementary Fig. 9f, g ) The findings above have shown that H3K56ac was involved in gene expression and there were enhanced H3K56ac around HPIP DNA-binding regions. H3K56ac was shown as a histone marks observed preferably during stress response at the replication forks, which was in line with our RNA-seq data from KO cartilage that showed cell death, DNA replication, and p53 pathway were significantly altered (Supplementary Tables 6 – 8 ), we then tested the possible connection of HPIP KO- H3K56ac in DNA replication and stresses response and its role in OA progression. The results indicated that HPIP KO diminished the recruitment ability of H3K56ac to the promoters of DNA replication and stresses response genes, which were derived from RNA-seq data (Supplementary Fig. 10a–f ). As HPIP is overexpressed in OA and HPIP causes increased H3K56 status in human OA chondrocytes, we next examined the relationship among the expression of H3K56ac , HPIP and LEF1 . The results showed that the level of HPIP expression was positively correlated with H3K56ac or LEF1 protein expression. Besides, H3K56ac expression was also positively associated with LEF1 protein expression (Supplementary Fig. 10g–k ). Taken together, these data demonstrate that HPIP directly activates expression of key Wnt signaling pathway targets by acetylating H3K56ac in their promoters in OA and HPIP had a crucial role in the OA progression. In the present study, we identified increased HPIP expression levels during OA progression. HPIP deficiency in mice impairs articular cartilage development and prevents the development of OA. Importantly, an intra-articular injection of AAV carrying a HPIP -specific shRNA showed protective effects against OA. The molecular network around HPIP was demonstrated at the molecular, cell, histological, functional, and clinical levels. Mechanistically, we found that HPIP physically binds to Wnt signaling transcriptional factors ( LEF1 ). Furthermore, HPIP colocalizes with LEF1 and activates the transcriptional activity of LEF1 and acetylates H3K56ac in the promoters of Wnt signaling pathway targets to modulate OA pathogenesis and HPIP expression is positively correlated with H3K56ac or LEF1 protein expression, suggesting that HPIP might be a promising therapeutic target against OA. HPIP was originally identified in a yeast two-hybrid screen as a PBX1 -binding protein [26] , and was shown to function as a corepressor of this transcription factor. HPIP participates in proliferation and progression. Our previous study revealed that HPIP regulates HBV X protein (HBx)-expressing hepatocarcinoma cell growth, invasion, EMT and metastasis through the AKT/mTOR or ERK/mTOR pathway [16] . In addition, HPIP interacts with casein kinase 1α ( CK1 α) and predicts the clinical outcomes for renal carcinoma [27] . HPIP also facilitates gastric cancer cell proliferation through activation of G1/S and G2/M cell cycle transitions and modulates colorectal cancer progression through activation of the MAPK/ERK1/2 and PI3k/AKT pathways [17] , [28] . Moreover, HPIP upregulation has been found in lung cancer [29] , [30] , ovarian cancer [31] , [33] , [33] , breast cancer [18] , [34] , thyroid cancer [35] , spinal glioblastoma [36] , head-and-neck squamous cell carcinoma [37] , and oral squamous cell carcinoma [38] , which indicates that HPIP is an important essential mediator in tumorigenesis. However, the exact role of HPIP in OA pathogenesis remains unknown. In the present study, we found that HPIP expression was significantly higher in OA cartilage. HPIP promoted the cell proliferation in chondrocytes. To characterize the specific functions of HPIP in cartilage development, we generated the chondrocyte-specific HPIP KO mice ( Col2a1-CreER T2 /HPIP f/f mice) and the mice revealed defects in bone development and proportional dwarfism compared to wild-type littermates. Similar observations that the cartilage specific cKO mice affect bone formation could also be found in other previous studies, such as Kdm6b cKO [15] , Rac cKO and Cdc42 cKO mice [39] . We speculated that the phenomenon might be related to the following reasons. First, the skeleton is mostly formed through the process of cartilage replacement in the growth plates of bones in a series of distinct chondrocyte differentiations steps, therefore, cartilage defects affect bone formation. Second, RNA-seq analysis suggested that HPIP could regulate a set of makers associated with ECM organization and skeletal system development. Disorganized structure of ECM also affects abnormal skeletal system development. In terms of PBX1 , as a transcription factor, PBX1 possesses the characteristics of activation or repression regulatory ability. Gordon et al. [24] reported that PBX1 repressed osteoblastogenesis by blocking Hoxa10 -mediated recruitment of chromatin remodeling factors. However, Selleri et al. [26] reported that PBX1 homozygous knockout mice revealed several defects in skeletogenesis, suggesting that PBX1 is required for bone formation and skeletal patterning. Moreover, Cheung et al. [40] reported that silencing of PBX1 decreased expression of Runx2 and Osterix , the two indispensable factors required for osteogenesis, indicating PBX1 has the cooperative function in osteogenesis. PBX1 protein is unable to activate or repress transcription alone [41] , but has to bind to other partner proteins including histone modification enzymes to exhibit the transcriptional function. The activation or repression function of PBX1 can be dependent on the type of histone modification enzymes it binds to and the type of bone-related gene promoters it recruits to. In the present study, we found PBX1 regulated osteogenesis. The detailed mechanisms underlying the PBX1 -mediated regulation in osteogenesis remain to be further elucidated. To further assess the structure of tibial subchondral bone, we performed the μCT and histology assay. Our histology results and bone tissue volume data obtained from μCT demonstrated that the subchondral bone plate (SBP) thickened in response to OA and cKO of HPIP led to decreased subchondral plate thickness and volume after surgery. The subchondral bone tissue volume of μCT data was in line with the histology findings, which is consistent with what we have expected. Moreover, we reported that the HPIP ablation genetic model could protect against developing OA. According to the combination of μCT and histopathological analysis, an intra-articular injection of AAV carrying HPIP -specific shRNA in C57BL/6J wild-type mice after ACLT surgery showed a protective effect against OA cartilage degradation, which supports HPIP ’s role as a potential clinical therapeutic candidate for OA treatment. To investigate the molecular mechanisms underlying the function of HPIP in OA, we performed RNA-Seq analysis to search for HPIP -mediated downstream target genes. We found a total of 1271 DEGs between the control and HPIP KO chondrocytes, including over 400 previously reported OA-associated genes [19] , [20] , [21] , [42] , [44] , [45] , [46] , [47] , [48] , [49] , [50] , [50] , which suggests that HPIP is closely related to the pathogenesis of OA. Moreover, HPIP -deficient chondrocytes were also found to exhibit decreased expression of CD9 , DCN , EPAS1 , FMOD , and SMURF2 , which have been reported to be inducers of OA. CD9 deficiency mice show a reduced severity of hallmarks of OA, including less cartilage degradation and soft tissue inflammation [19] . DCN -deficient mice develop significantly less OA after forced exercise than wild-type mice [20] . EPAS1 -deficient mice show resistance to OA development [46] . The Bgn/FMOD double-deficient mouse demonstrates an increase in bone and subchondral bone volume as well as in the expression of collagen type X and aggrecan compared with wild-type controls [48] . SMURF2 has been reported to cause spontaneous OA in mice [43] . Our study showed that HPIP is as an upstream regulator of these five known critical OA inducers ( CD9 , DCN , EPAS1 , FMOD , and SMURF2 ), extending our understanding of the importance of HPIP in OA regulation. Moreover, we identified that HPIP -deficient mice protect against developing OA. Importantly, the intersection of ChIP-seq and RNA-seq data indicated that HPIP-modulated OA pathogenesis through regulation of Wnt signaling. The Wnt signal transduction pathway is an important main regulator of development and disease [51] , [53] , [53] . The Wnt signaling pathway controls normal aging and contributes to human OA [54] , [56] , [56] . In this study, we found that HPIP deficiency in OA chondrocytes impaired Wnt signaling. Subsequent analysis demonstrates that HPIP exerts its biological function mainly through interactions with transcriptional factors ( LEF1 ) to activate Wnt signaling. LEF1 is a sequence-specific DNA-binding protein which is expressed in adult mice pre-B and T lymphocytes and in the mesencephalon, neural crest, whisker follicles, tooth germs, and other sites during the progression of embryogenesis [57] , [58] . Previous reports have shown that LEF1 -null mice exhibit developmental defects in teeth, hair follicles, mammary glands, and the brain [58] . Besides, in terms of skeletal metabolism, analysis of LEF1 -null mice is hampered by their perinatal lethality [59] . In the present study, we also found LEF1 knockdown inhibited the proliferation of chondrocytes, which was in line with the previous findings. HPIP inhibition results in marked suppression of recruitment of H3K56ac to the promoters of Wnt target genes. H3K56ac was shown to be a histone marks observed preferably during stress response at the replication forks, which was in line with our RNA-seq data from KO cartilage that showed cell death, DNA replication, and p53 pathway were significantly altered. In the present study, we also found HPIP KO diminished the recruitment ability of H3K56ac to the promoters of DNA replication and stresses response genes. Besides, H3K56ac expression was also positively correlated with HPIP and LEF1 protein expression, revealing a molecular network around HPIP , LEF1 , and H3K56ac dynamics and Wnt signaling in OA. Collectively, our findings demonstrated that HPIP expression was increased in OA. HPIP deficiency in mice impairs articular cartilage development and protects against developing OA. An intra-articular injection of AAV carrying HPIP -shRNA in vivo attenuated OA articular cartilage degradation when administered after injury. Mechanistically, we showed that HPIP physically interacts with LEF1 to promote transcription of Wnt target genes. HPIP potentiates LEF1 transcriptional activity and acetylates H3K56ac around Wnt signaling target gene promoters, thus suggesting that HPIP may be an attractive therapeutic target for treating OA patients. Further investigation is warranted to evaluate the efficacy of lentivirus encoding HPIP -specific shRNA in OA models of large animals before the clinical trials. 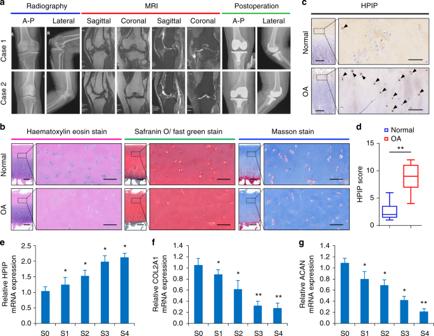Patients and specimens All human studies were conducted with informed consent of the patients and approval of the Institutional Ethics Review Board of the General Hospital of the People’s Liberation Army (Beijing, China). OA was macroscopically diagnosed according to the Modified Outerbridge Classification [60] , [61] (stage 0, intact cartilage; stage 1, chondral softening and or blistering with intact surface; stage 2, superficial ulceration, fibrillation, or fissuring < 50% of depth of cartilage; stage 3, deep ulceration, fibrillation, fissuring, or chondral flap > 50% of cartilage without exposed bone; and stage 4, full-thickness wear with exposed subchondral bone). Articular cartilage samples were collected from 118 patients with knee OA who underwent knee arthroplasty surgery. Specimens that included all cartilage layers and subchondral bone were separately harvested from sites on the tibial plateau by drilling holes (4.5 mm). Clinical information was collected from patient records. Fig. 1 HPIPexpression is upregulated in osteoarthritis (OA) cartilage.aRepresentative plain radiographs and MRI images of patients with knee OA undergoing knee arthroplasty surgery. A–P anterior–posterior.bRepresentative histopathological staining of normal and OA cartilage tissues. Hematoxylin–eosin, safranin O/fast green and Masson trichrome staining were performed to examine the proteoglycan content in cartilage. Scale bar, left, 500 μm; right, 200 μm.cImmunohistochemistry assay with anti-HPIPin normal and OA cartilage tissues. Scale bar, left, 500 μm; right, 50 μm.dTheHPIPscores in normal (n= 118) and OA (n= 118) cartilage tissues based on an immunohistochemistry assay were compared with the Mann–WhitneyU-test. Center value represents the median of theHPIPscores. The bounds of box represent the upper quartile and the lower quartile. The whiskers represent the maximum and minimum score.eqRT-PCR measurement ofHPIPin cartilage tissues obtained from stage 0 (S0) to stage 4 (S4).fqRT-PCR measurement ofCOL2A1in cartilage tissues obtained from stage 0 (S0) to stage 4 (S4).gqRT-PCR measurement ofACANin cartilage tissues obtained from stage 0 (S0) to stage 4 (S4). Error bar represents the standard deviation (s.d.) andP-value was generated by using one-way ANOVA with Tukey’s post hoc test. *P< 0.05; **P< 0.01 The clinical and demographic characteristics of the study population are shown (Supplementary Table 1 ). Mice HPIP f/f mice were generated by Cyagen Biosciences Inc. Col2a1-CreER T2 mice (Stock Number: 006774) were obtained from Jackson Laboratories (Bar Harbor, ME, USA). Both HPIP f/f and Col2a1-CreER T2 mice were in a C57BL/6J background. To generate Col2a1-CreER T2 ; HPIP f/f mice, HPIP f/f mice were mated with Col2a1-CreER T2 mice to obtain Col2a1-CreER T2 ; HPIP f/+ mice, which were then mated with HPIP f/f mice. HPIP general knockout mice were generated by Shanghai Model Organisms Center, Inc using CRISPR/Cas9. The guide RNA targeting exon 3 of HPIP gene was designed. The guide RNA sequence is TGGAGGAGTCCCGAAGGGCCTGG. The exon 3 region in HPIP is from 225 to 247. A mixture of plasmids encoding Cas9 and HPIP guide RNA was microinjected into the fertilized C57BL/6 eggs, and the transgenic embryos were planted into pseudopregnant recipients. Founder lines of successful mutation of the HPIP gene cluster were identified through PCR genotyping of tail DNA. The positive female founder mice and wild-type male mice were bred to get F1 HPIP heterozygote mice. Male HPIP heterozygote mice and female HPIP heterozygote mice were then crossed to obtain HPIP homozygote mice. For mouse embryo genotype identification, genomic DNA was prepared from the tail tips of 14-day-old embryos and the HPIP mutation was identified by PCR amplification, DNA sequencing and immunoblot. All mice used in the OA evaluation were males to avoid any potential postmenopausal bone loss effect and were maintained under pathogen-free conditions. All experimental procedures were approved by the Institutional Animal Care and Research Advisory Committee of the General Hospital of the People’s Liberation Army. ACLT surgery Eight-week-old Col2a1-CreER T2 ; HPIP f/f mice and their HPIP f/f littermates were injected intraperitoneally with tamoxifen (Sigma, St. Louis, MO, USA; 100 μg/g body weight) daily for 5 days before surgical induction of OA. We anesthetized the mice from this group with ketamine and xylazine and then underwent ACLT surgical transection of the right knee to induce mechanical instability and create an experimental OA model. Sham operations were performed on control mice. We analyzed Col2a1-CreER T2 ; HPIP f/f mice and their HPIP f/f littermates 4 and 8 weeks after surgery. Investigators were blinded to the genotype of the mice when surgical transection was performed. The OARSI system (grades 0–6) was used to quantify OA severity, which was also evaluated by observers who were blinded to the experimental group. Cell culture Normal chondrocytes were obtained from the knees of patients who had died of diseases unrelated to arthritis. Arthritic chondrocytes were obtained from patients undergoing elective total knee arthroplasty for end-stage OA according to a modified Outerbridge scale (Grade III: maximal fibrillation). The chondrocytes were incubated in high glucose Dulbecco’s modified Eagle’s medium (DMEM) with 10% fetal calf serum (FCS), 100 IU/ml penicillin and 100 μg/ml streptomycin at 37 °C in an atmosphere of 5% CO 2 . The characterization of the chondrocyte phenotype was established through the analysis of COL2/COL1 gene expression. First-passage chondrocytes at 85% confluence were used for all experiments. HPIP knockout chondrocytes HPIP knockout (KO) chondrocytes were generated by CRISPR/Cas9 (Santa Cruz Biotechnology, Inc.). The CRISPR/Cas9 KO Plasmid (sc-412788) and the control CRISPR/Cas9 Plasmid (sc-418922) infection for HPIP were performed according to the manufacturer’s instructions. Briefly, the Plasmid DNA solution was added directly to the dilute UltraCruz® Transfection Reagent (sc-395739) using a pipette, and incubated for 30 min at room temperature. Then the chondrocytes were incubated for 24–72 h under conditions normally used to culture the cells. The KO efficiency of HPIP in chondrocytes was then confirmed by western blotting. RNA-sequencing analysis Isolated HPIP KO and the control chondrocytes were filtered through 70 mM nylon filters (BD), washed twice with sterile PBS, and then were directly prepared for cDNAs amplification and RNA-Seq library construction without any culture. Total RNA was isolated with TRIzol reagent from HPIP KO and the control chondrocytes. A complementary DNA library was prepared and sequencing was performed according to the Illumina standard protocol by Beijing Novel Bioinformatics Co., Ltd. ( https://en.novogene.com/ ). Raw reads from RNA-seq libraries were trimmed to remove the adaptor sequence and the reads with adaptor contaminants and low-quality reads (the mass value Q -score < 5 of the base number accounts for more than 50%) and reads from N ( N indicates that the base information that cannot be determined) which is >10%. After filtering, reference genome and gene model annotation files were downloaded from a genome website browser (NCBI/UCSC/Ensembl). Indexes of the reference genome were built using Bowtie v2.0.6 and paired-end clean reads were aligned to the reference genome using TopHat v2.0.9. Bowtie was used for a BWT (Burrows–Wheeler Transformer) algorithm for mapping reads to the genome and Tophat can generate a database of splice junctions based on the gene model annotation file and thus achieve a better mapping result than other non-splice mapping tools. For the quantification of gene expression level, HTSeq V0.6.1 was used to count the read numbers mapped for each gene. The RPKM of each gene was calculated based on the gene read counts mapped to this gene. A differential expression analysis was performed using the DESeq R package (1.10.1). For clustering, we clustered different samples to see the correlation using hierarchical clustering distance method with the function of heatmap, SOM (Self-organization mapping) and kmeans using silhouette coefficient to adapt the optimal classification with default parameter in R. The RNA-seq data in this study was deposited at Gene Expression Omnibus (GEO) ( http://www.ncbi.nlm.nih.gov/geo/ ) under accession ID GSE100312. ChIP-sequencing assay A ChIP assay was performed using a commercially available kit (Millipore, MA, USA) [62] . One hundred nanograms of DNA fragments were used per ChIP. Sequencing libraries were prepared from collected HPIP ChIP and corresponding input DNA by blunting, A-tailing and adaptor ligation using NEXTFlex barcoded adapters (Bioo Scientific). Libraries were PCR-amplified for 16 cycles, fragments with size of 300 bp were processed using the Covaris Focused-ultrasonicators (Covaris, Inc. S220). Sequencing was performed using the Hi-Seq 2500 (Illumina) platform at Beijing Novel Bioinformatics Co., Ltd. ( https://en.novogene.com/ ). ChIP-seq data were aligned to the hg19 genomes using bowtie-0.12.9. The basic quality statistics analysis of raw reads was evaluated by the FastQC software. Raw reads were then trimmed to remove the duplicate reads and reads that were matched with the adaptor sequence and the base whose mass value of the 3′-tail base number that was <20. If the remaining sequence length was not shorter than 18 nt, it will be retained. Only tags mapped uniquely to the genome were considered for further analysis. We select 13 as the threshold for mapping quality (MAPQ) to ensure the high quality. Genomic binding peaks for HPIP were identified using the findPeaks command from HOMER ( http://homer.salk.edu/homer/ ) with eightfold enrichment over the input sample. Peaks were annotated using the annotatePeaks command. HPIP -related transcription factor binding motifs were performed with command findMotifsGenome.pl. The complete ChIP-seq datasets in this study was deposited at GEO database ( http://www.ncbi.nlm.nih.gov/geo/ ) under accession ID GSE100312. Gene ontology (GO) and KEGG enrichment analysis GO enrichment analysis of differentially expressed genes was implemented by the GOseq R Package, in which gene length bias was corrected. GO analysis was performed with the DAVID online tool ( https://david.ncifcrf.gov/ ). Top GO categories were selected according to the P -values. Pathways of differentially expressed genes were analyzed by the KEGG database ( http://www.kegg.jp/kegg/ ). We used KOBAS software to test the statistical enrichment of differential expression genes in KEGG pathways. Adeno-associated virus (AAV) The AAV vector was generated after cloning short hairpin RNA (shRNA) fragments into the adeno-associated virus vector GV478 (Shanghai Genechem Co., Ltd). AAV packaging was performed by cotransfecting AAV-293 cells with the recombinant AAV vector, pAAV-RC vector, and pHelper vector. AAV were collected from the AAV-293 cell supernatant, condensed, and purified for further animal experiments. Intra-articular administration C57BL/6J wild-type mice were anesthetized with 3% isoflurane and maintained with a 2% isoflurane and oxygen mixture, and then, the skin above the articular joint was shaved. Adeno-associated virus carrying HPIP -specific shRNA was produced as described above. Virus-containing medium was collected and passed through a 0.45 μm filter (Millipore) to remove cell debris. Then, the adeno-associated virus of the supernatant was concentrated by ultracentrifugation at 28,800 × g at 4 °C for 2 h. The supernatant was subsequently discarded, and the precipitate was resuspended in 100 ml PBS. Mice were injected intra-articularly with this solution using 33-gauge needles (Hamilton Company) and 25 µl CASTIGHT syringes (Hamilton Company). Rotarod and hotplate analysis Unanesthetized mice were put onto an accelerating rotarod (Ugo Basile). Briefly, the first round time was recognized by the duration to stay atop the rod for the first failure. Mice at different time points after surgery were randomly assigned into different groups. Each trial had a maximum time of 5 min. Mice were given an intertribal rest interval of 30 min. For hotplate analysis, unanesthetized mice of different groups were put on the 55 °C hotplate (Columbus Instruments). Time of response (jumping, licking, or jumping) for the latency period was recorded. Rotarod and hotplate analysis were evaluated by observers who were blinded to the experimental group. Pain measurement Pain behaviors were assessed as hind limb weight-bearing asymmetry. Weight-bearing asymmetry was measured as the difference between hind limbs as a percentage of total weight borne through both hind limbs [63] , [64] . Mice were acclimated to the test room for 30 min before open field testing [65] . Mice were placed in the center of individual plexiglass square chambers (45 cm × 45 cm) and allowed to freely explore the chamber for the duration of the 6-min test session. The movements of the mice were recorded with a video camera. Upon completion of the test, which was performed once per animal, each mouse was returned to its home cage. Two observers blinded to treatment group assignments manually traced mouse movements to calculate the distance (in cm) that the mouse traveled within the cage in 6 min (traveled distance). μCT analysis Mouse knee joints were harvested, and soft tissues including muscles and skins were dissected. The remaining tissues were including the whole original mouse knee joints were fixed in formaldehyde and then were stored in 70% ethanol. CT scanning was performed using high resolution μCT (Skyscan 1172). Images were analyzed and reconstructed with CTAn v1.9 and NRecon v1.6. Three-dimensional model visualization software (CTVol v2.0) was also used. A voltage of 50 kVp, a resolution of 5.7μm per pixel and a current of 200 μA were set for the scanner. The transverse, coronal and sagittal images of the knee joints were used for analyses. The region of interest covering the surface area of tibia was collected. After scanning, each sample was assigned a random number for ensure blinded assessment, and then was processed for the image processing. The transverse, coronal and sagittal images of the knee joints were used for analyses. The region of interest covering the surface area of tibia was collected. After scanning, each sample was assigned a random number for ensure blinded assessment, and then was processed for the image processing. Histology and immunohistochemical assay Cartilage tissues were fixed in 4% buffered paraformaldehyde for 48 h and subsequently decalcified with buffered EDTA (20% EDTA, pH 7.4). The tissues were embedded in paraffin, sectioned and stained with hematoxylin–eosin (HE), safranin O/fast green and Masson’s trichrome. The thickness of the medial subchondral bone plate (region between the osteochondral junction and marrow space on the medial side of the tibial plateau, in μm) was measured in a blinded fashion with OsteoMeasureXP Software (OsteoMetrics, Inc.). The histopathological changes were blindly scored using the modified Mankin grading system. For whole skeleton staining, mice were collected, and the soft tissues of skin, viscera, and adipose tissue were removed and then fixed in 95% (v/v) ethanol for 1 week. The specimens were then transferred to acetone and stained in a solution containing Alizarin red S and Alcian blue 8GX (Sigma-Aldrich) at 37 °C, protected from light. The rinse the mice in 1% aqueous KOH for 2 days. The specimens were stored in 100% glycerol. Immunohistochemical assay was performed using a standard protocol. Briefly, the articular cartilage sections were pre-treated for 10 min with trypsin (0.05%) prior to treatment with 3% (vol/vol) H 2 O 2 for 15 min. Subsequently, the sections were blocked with 10% goat serum for 1 h at room temperature. After washing with PBS, primary antibodies (anti-Collagen II, 1:100, Abcam, ab34712; anti-Aggrecan, 1:50, Abcam, ab36861) were applied to the sections and incubated overnight at 4 °C. The sections were subsequently washed with PBS and incubated for 15 min with biotinylated secondary antibody, followed by incubation for 30 min using the Histostain Plus kit (Invitrogen). Lastly, the sections were washed and incubated for 2 min with 3, 3′-diaminobenzidine (DAB) substrate. Using light microscopy, two experienced pathologists blindly reviewed the stained tissue sections. The widely accepted German semi-quantitative scoring system [66] , considering the staining intensity and area extent: 0, negative staining; 1, weakly positive staining; 2, moderately positive staining; and 3, strongly positive staining; The extent of marker expression was quantified by evaluating the percentage of the positive staining areas in relation to the whole area in the core. In addition, a score of 0 (<5%), 1 (5–25%), 2 (25–50%), 3 (51–75%), and 4 (>75%) were given for the reactivity. The final immunoreactive score was determined by multiplying the intensity and the extent scores, yielding a range from 0 to 12. For the assay, we defined a 0 score as negative and scores of 1-12 as positive. Plasmids For the eukaryotic expression vectors encoding FLAG -, MYC -fusion proteins tagged at the amino terminus were constructed by inserting PCR-amplified fragments into pcDNA3 (Invitrogen) or pIRESpuro2 (Clontech). LEF1 -response element (LRE) promoter luciferase reporters were generated through insertion of PCR-amplified promoter fragments from genomic DNA into the pGL4 -basic vector (Promega). Lentiviral shRNA vectors were generated after cloning short hairpin RNA (shRNA) fragments into the lentiviral vector pSIH-H1-Puro (System Biosciences). Lentiviruses were produced through cotransfection of HEK293T cells (RRID:CVCL_0063) with recombinant lentivirus vectors and the pPACK Packaging Plasmid Mix (System Biosciences) using a Megatran reagent (Origene). Lentiviruses were collected at 48 h after transfection and added to the medium of target cells with 8 μg/ml Polybrene (Sigma-Aldrich). Plasmids encoding GST-fusion proteins were prepared by cloning into pGEX-KG (Amersham Pharmacia Biotech). For the yeast two-hybrid assay, the bait plasmid pAS2-LEF1 was constructed by inserting the full-length LEF1 cDNA fragment into pAS2-1 (Clontech). Details of the cloning are available upon request. Quantitative reverse-transcription PCR (qRT-PCR) Total RNA was extracted and reverse-transcribed into cDNA using a RNeasy Mini kit (Qiagen) according to the manufacturer’s instructions. Expression of mRNAs was determined using SYBR Premix Ex Taq Master Mix (2×) (Takara). The relative expression level of the target was calculated using the comparative Ct method. β-actin was used as an internal control to normalize sample differences. The sequences of the primers used for qRT-PCR analysis are presented (Supplementary Table 10 ). Western blotting Total proteins were extracted from tissues or chondrocytes using RIPA buffer (50 mM Tris–HCl (pH 7.4), 150 mM NaCl, 20 mM EDTA, 1% Triton X-100, 1% sodium deoxycholate, 1% SDS and protease inhibitors, Wheaton Science) on ice for 30 min and analyzed using SDS-PAGE electrophoresis. Membranes were incubated with anti- HPIP (1:50, Proteintech, 12102-1-AP), anti- LEF1 (Abcam, 1:200, ab137872), anti- CCND1 (Abcam, 1:2 000, ab134175), anti- c-Myc (Abcam, 1:1 000, ab32072), anti- CUL1 (Abcam, 1:200, ab75817), anti- WNT9A (Abcam, 1:100, ab125957), anti- FZD1 (Abcam, 1:50, ab71342), anti- LRP5 (Abcam, 1:50, ab36121). Immunocomplexes were visualized through chemiluminescence using an ECL kit (Amersham Biosciences). Uncropped scans of the most important immunoblots are shown in Supplementary Information (Supplementary Fig. 11 ). Cell adhesion assay For the adhesion assay, a 96-well plate was coated with fibronectin (Sigma) as the manufacturers’ instructions. Wells were blocked for 30 min with 0.5% heat-inactivated BSA/PBS, rinsed three times with PBS. HPIP KO and the control chondrocytes were seeded and incubated at 37 °C for 40 min. After washing with serum-free media, adherent cells were fixed, stained and solubilized for absorbance measurement (650 nm). Migration and cell growth assays Cells were seeded in 6-well plates at 70% confluence in culture medium for migration assays [67] . After 24 h, the confluent cellular monolayer was scratched with a fine pipette tip. For migration, the rate for migration was observed at the indicated times using a microscope. For cell growth, cell proliferation was assessed by using a CCK-8 Kit (Dojindo Laboratories, Kumamoto, Japan) according to the manufacturer’s instructions. Chondrocytes were seeded in 96-well plates and examined at 0, 24, 48, 72, and 96 h. Yeast two-hybrid assay The bait plasmid pAS2-LEF1 and a human mammary two-hybrid cDNA library (Clontech) were sequentially transformed into Saccharomyces cerevisiae strain CG1945 according to the manufacturer’s instructions (Clontech). Transformants were grown on synthetic medium lacking tryptophan, leucine, and histidine but containing 1 mM 3-aminotriazole. Approximately one million transformants were screened. The candidate clones were rescued from yeast cells and re-transformed into the same yeast strain to verify the interaction between the candidates and bait. The specificity of the interaction was examined by comparing the interactions between the candidates and various bait constructs. The unrelated bait plasmid pAS2-lamin C was used as a negative control. Subcellular fractionation The localization of proteins was examined by subcellular fractionation. Briefly, cells were homogenized using a Dounce homogenizer, and the homogenate was centrifuged at 366 × g for 10 min. The pellet was then analyzed as the nuclear fraction. The supernatant was centrifuged again at −16,200 × g for 10 min, and the final supernatant was analyzed as the cytoplasmic fraction. Chromatin immunoprecipitation (ChIP) assay and re-ChIP ChIP assay was performed using the Magna ChIP Assay Kit (Millipore) according to the manufacturer’s instructions [68] . Three million chondrocytes were fixed in 37% formaldehyde, pelleted, and resuspended in lysis buffer. The cells were sonicated and centrifuged to remove insoluble material. The supernatants were collected, and protein G magnetic beads were added and incubated for 1 h at 4 °C with anti- HPIP (Proteintech, 1:50, 12102-1-AP), anti- LEF1 (Abcam, 1:50, ab137872), H3K4ac (Abcam, 1:50, ab176799), H3K9ac (Abcam, 1:50, ab10812), H3K14ac (Abcam, 1:50, ab52946), H3K56ac (Abcam, 1:25, ab71956). The chromatin was collected, purified, and de-crosslinked at 62 °C for 2 h, followed by incubation at 95 °C for 10 min. The DNA was isolated using the ChIP DNA Clean & Concentrator kit (Zymo Research Corp.) according to the manufacturer’s instructions. The precipitated DNA fragments were quantified through RT-PCR analysis. For re-ChIP, complexes were eluted from the primary immunoprecipitation by incubation with 10 mM DTT at 37 °C for 30 min and diluted 1:50 in re-ChIP buffer (150 mM NaCl, 1% Triton X-100, 2 mM EDTA, 20 mM Tris–HCl, pH 8.1) followed by re-immunoprecipitation with the second antibodies. RT-PCR was performed to detect relative occupancy. GST pull-down and coimmunoprecipitation assays For the GST pull-down assay, GST-fusion proteins were expressed and purified according to the manufacturers’ instructions (Amersham Pharmacia and Qiagen). Cell lysates expressing target proteins were incubated with GST-fusion proteins bound to GST beads (Amersham Pharmacia), and the pull-down proteins were examined. For the coimmunoprecipitation assay, cells were harvested and lysed in lysis buffer on ice for 30 min. After centrifugation at 4 °C at 13,800 × g for 15 min, antibodies were added to the supernatant with rolling at 4 °C overnight. Protein G or A agarose (Santa Cruz) was then added to the samples, and the samples were rolled at 4 °C for 2 h. After the beads were washed three times with lysis buffer, the pellets were dissolved into 2 × SDS loading buffer after centrifugation and boiled at 100 °C for 10 min. Proteins were analyzed by immunoblotting with the indicated antibodies. Statistical analysis Statistical analysis of the RNA-seq data was performed, and a two-tailed t -test with the Benjamini and Hochberg correction was used. All data were log transformed. GO terms with corrected P -values <0.05 were considered significantly enriched by differentially expressed genes. Evaluation of quantitative RT-PCR data was performed using one-way ANOVA with Tukey’s post hoc test. All analyses were performed using SPSS software 17.0 or GraphPad PRISM 6 (GraphPad). The data are expressed as the mean ± standard deviation, and P < 0.05 was considered statistically significant.